Combinatorial targeting and discovery of ligand-receptors in organelles of mammalian cells Phage display screening allows the study of functional protein–protein interactions at the cell surface, but investigating intracellular organelles remains a challenge. Here we introduce internalizing-phage libraries to identify clones that enter mammalian cells through a receptor-independent mechanism and target-specific organelles as a tool to select ligand peptides and identify their intracellular receptors. We demonstrate that penetratin, an antennapedia-derived peptide, can be displayed on the phage envelope and mediate receptor-independent uptake of internalizing phage into cells. We also show that an internalizing-phage construct displaying an established mitochondria-specific localization signal targets mitochondria, and that an internalizing-phage random peptide library selects for peptide motifs that localize to different intracellular compartments. As a proof-of-concept, we demonstrate that one such peptide, if chemically fused to penetratin, is internalized receptor-independently, localizes to mitochondria, and promotes cell death. This combinatorial platform technology has potential applications in cell biology and drug development. For more than a decade, in vivo phage display has allowed identification of novel peptide ligands that selectively target blood vessels of normal organs or tissues and tumours [1] , [2] . Biochemical approaches such as affinity chromatography or genetic approaches such as similarity mining of online databases have subsequently identified the corresponding organ- and tissue-selective cell surface receptors for such ligands—discoveries which, in turn, have revealed novel roles for known proteins and identified additional proteins that are differentially expressed in the vasculature of normal and pathologic tissues [3] , [4] , [5] . These endothelial surface receptors regulate sophisticated vascular functions as either tissue-specific or angiogenesis-related 'ZIP codes'. This combinatorial selection methodology also proved to be versatile when applied to the cell surface; indeed, the biological diversity at the cell membrane level can be probed even when cells have been removed from their usual tissue architecture. For example, using a single step-phase-separation technique [6] , we have ligand-profiled the membrane receptor diversity of the NCI collection of 60 human tumour cell lines and have classified these lines based on expression of their putative tumour cell surface receptor proteome [7] . Moreover, from a screen on white adipose tissue-derived stem cells, we have identified integrin α5β1 as a receptor for SPARC [8] , characterized a novel ternary complex involving netrin-4 that controls the migration and proliferation of neural stem cells [9] , discovered ligand motifs that target the macropinocytotic pathway in leukaemia cells [10] , and defined a supramolecular complex, the 'leukaemia cell invadosome', which is essential for the pericellular proteolysis and migratory capacity of acute myelogenous leukaemia cells [11] . Recently, we have generated prototype drugs for the vascular endothelial growth factor and epidermal growth factor pathways [12] , [13] , and have developed phage-based hydrogels for three-dimensional tissue culture based on magnetic cell levitation [14] . Whereas phage library screening in vitro and in vivo has consistently uncovered novel protein–protein interactions at the cell surface, the technology has not yet enabled direct and straightforward targeting of intracellular organelles and signal transduction or metabolic pathways. Currently, intracellular ligand-directed delivery can be accomplished by supercharged proteins or cell-penetrating peptides that induce receptor-independent crossing of eukaryotic cell membranes; such peptides are usually arginine-rich cationic sequences [15] , [16] , [17] , [18] , [19] . One of the best characterized of these peptides is penetratin (pen), a motif derived from the third helix of the homeodomain of Drosophila antennapedia protein [20] , [21] , [22] . The mechanism of pen internalization is energy-dependent, lipid-raft-mediated endocytic uptake [23] . Pen has previously been used to transport peptides, recombinant proteins, antibodies, small interfering RNA, and micro RNA into cells [24] , [25] , [26] , [27] , [28] , [29] , [30] , [31] , [32] , [33] . Reports that certain cell-penetrating peptides, such as pen or human immunodeficiency virus type 1 Tat protein, improve cellular uptake of eukaryotic viruses (such as adenoviruses), and enable delivery of prokaryotic viral particles (such as λ phage) into mammalian cells [34] , [35] stimulated us to determine whether combinatorial phage display methodology could be adapted for the direct analysis of intracellular protein–protein interactions and to discover internalizing homing peptide (iHoPe) motifs affecting metabolic pathways. Here we introduce a new class of filamentous phage-based reagents that integrate pen [36] as a fusion protein with the recombinant major coat protein (rpVIII) and thereby enable receptor-independent phage particle entry into mammalian cells. Moreover, either random peptide libraries or specific individual motifs can be simultaneously displayed on the minor coat protein (pIII), a feature allowing both intracellular library selection and targeting of organelles. We have termed this new family of reagents 'internalizing phage' (iPhage). In this initial study, our central goal was to identify an intracellular targeted peptide that would induce programmed cell death as a biological surrogate readout and proof-of-concept for our general selection approach. Indeed, we have uncovered an iHoPe that induces cell death via ribosomal protein L29 (RPL29), and therefore demonstrate that the combinatorial selection of internalizing peptides is feasible. One hopes that future studies with this enabling platform technology will tackle other biological end points in disease-specific settings. Functional iPhage particles cross mammalian cell membranes The general structure of iPhage was generated on the backbone phage vector f88-4 (ref. 37 ; Fig. 1a ) displaying pen (sequence RQIKIWFQNRRMKWKK) on rpVIII ( Fig. 1b ). As controls, we used parental phage and site-directed mutant iPhage displaying a mutant loss-of-function form of pen (RQIKI A FQNRRMK A KK), in which two critical tryptophan (W) residues (required for membrane translocation) were mutated to alanine (A) residues ( Fig. 1c ). We observed abundant iPhage production in K91 Escherichia coli , indicating that iPhage constructs were correctly assembled and non-toxic to the host bacteria. 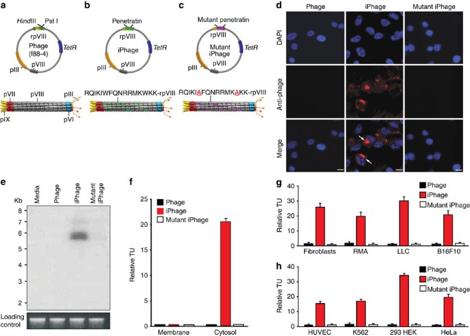Figure 1: Display of pen on rpVIII mediates receptor-independent cell internalization. (a) Upper: parental f88-4 phage vector contains two capsid genes encoding a wild-type (wt) protein VIII (pVIII, depicted in grey) and a recombinant protein VIII (rpVIII; depicted in green). The recombinant gene VIII contains a foreign DNA insert with aHindIII and aPstI cloning site (depicted in red).TetR, tetracycline resistance gene. Lower: representation of the assembled phage particle expressing only the wt major coat protein pVIII (grey); pIII, minor coat protein (orange); pVI protein (blue); pVII protein (red), and pIX protein (yellow). (b) Upper: annealed oligonucleotides encoding the pen peptide were cloned in frame with the recombinant gene VIII. Lower: iPhage particles displaying the pen peptide motif (RQIKIWFQNRRMKWKK) at the amino terminus of the rpVIII (green). (c) Upper: the mutant iPhage genome has nucleotide substitutions in the pen sequence replacing tryptophan (W) by alanine (A) residues (underlined in red). Lower: representation of the assembled mutant iPhage displaying mutant pen on rpVIII protein (purple). (d) Immunofluorescence of KS1767 cells shows internalized viral particles only in cells incubated with iPhage. The nuclear stain DAPI emits blue fluorescence, and internalized phage particles were detected with conjugated antibodies (red fluorescence). Scale bar, 100 μm. (e) Phage genomic DNA was detected only in KS1767 cells incubated with iPhage particles (Southern blot, upper panel). Total genomic DNA stained with ethidium bromide served as a loading control (lower panel). (f) iPhage particles are internalized and viable in the cytosol and undetected in the membrane fraction of KS1767 cells. Bars represent mean values for TU recovered from the cytosol±s.e.m., from triplicates. Phage internalization by various types of cultured cells (g) mouse and (h) human. RMA (Rauscher murine leukaemia virus antigen) lymphoma, LLC (Lewis lung carcinoma), B16F10 (Melanoma), HUVEC (human umbilical vein endothelial cell), leukaemia (K562), 293HEK (human embryonic kidney) and HeLa cell lines. Internalization assays were run in triplicate; bars represent mean values for phage TU recovered from the cytosol-enriched fraction±s.e.m. from triplicates. Figure 1: Display of pen on rpVIII mediates receptor-independent cell internalization. ( a ) Upper: parental f88-4 phage vector contains two capsid genes encoding a wild-type (wt) protein VIII (pVIII, depicted in grey) and a recombinant protein VIII (rpVIII; depicted in green). The recombinant gene VIII contains a foreign DNA insert with a Hind III and a Pst I cloning site (depicted in red). TetR , tetracycline resistance gene. Lower: representation of the assembled phage particle expressing only the wt major coat protein pVIII (grey); pIII, minor coat protein (orange); pVI protein (blue); pVII protein (red), and pIX protein (yellow). ( b ) Upper: annealed oligonucleotides encoding the pen peptide were cloned in frame with the recombinant gene VIII. Lower: iPhage particles displaying the pen peptide motif (RQIKIWFQNRRMKWKK) at the amino terminus of the rpVIII (green). ( c ) Upper: the mutant iPhage genome has nucleotide substitutions in the pen sequence replacing tryptophan (W) by alanine (A) residues (underlined in red). Lower: representation of the assembled mutant iPhage displaying mutant pen on rpVIII protein (purple). ( d ) Immunofluorescence of KS1767 cells shows internalized viral particles only in cells incubated with iPhage. The nuclear stain DAPI emits blue fluorescence, and internalized phage particles were detected with conjugated antibodies (red fluorescence). Scale bar, 100 μm. ( e ) Phage genomic DNA was detected only in KS1767 cells incubated with iPhage particles (Southern blot, upper panel). Total genomic DNA stained with ethidium bromide served as a loading control (lower panel). ( f ) iPhage particles are internalized and viable in the cytosol and undetected in the membrane fraction of KS1767 cells. Bars represent mean values for TU recovered from the cytosol±s.e.m., from triplicates. Phage internalization by various types of cultured cells ( g ) mouse and ( h ) human. RMA (Rauscher murine leukaemia virus antigen) lymphoma, LLC (Lewis lung carcinoma), B16F10 (Melanoma), HUVEC (human umbilical vein endothelial cell), leukaemia (K562), 293HEK (human embryonic kidney) and HeLa cell lines. Internalization assays were run in triplicate; bars represent mean values for phage TU recovered from the cytosol-enriched fraction±s.e.m. from triplicates. Full size image To demonstrate that iPhage can cross mammalian cell membranes through a receptor-independent mechanism, we exposed human Kaposi sarcoma (KS) 1767 cells to each of the three individual constructs. After 24 h, phage particles were detected in cells exposed to iPhage but not in cells incubated with either parental phage or mutant iPhage ( Fig. 1d ). In addition, phage genomic DNA was detected only in cells infected with iPhage particles suggesting that all viral components were internalized ( Fig. 1e ). Furthermore, pre-incubation of the soluble pen peptide on mammalian cells did not block iPhage particle internalization, a result indicating that the intracellular uptake is receptor-independent and non-saturable ( Supplementary Fig. S1 ). To test viability and eliminate the possibility that iPhage particles have either affinity or get trapped in the cell surface; we isolated plasma membrane and cytosol fractions and recovered the viral pool by infection of host E . coli ; a marked recovery of viable iPhage particles were observed in the cytosol after 24 h, in comparison to parental phage and mutant iPhage that served as negative controls ( Fig. 1f ). We did not recover parental phage, iPhage, or mutant iPhage from the membrane fraction, a result indicative that phage particles were not nonspecifically trapped within the cell surfaces. Moreover, to account for a possible uptake of iPhage particles by endocytosis, we have performed a series of co-localization studies with markers of early (EEA1) and late (mannose 6-phosphate receptor) endosomes. Careful analysis of serial confocal images demonstrated that, on cellular intake, iPhage particles do not totally reside in the endosomal compartment but rather, are evenly distributed in the cytosol. Notably, additional co-immunostaining studies with markers of intracellular organelles such as Golgi apparatus and mitochondria confirmed these findings; iPhage particles showed a random intracellular distribution according to different subcellular markers detected by confocal microscopy (that is, Golgi apparatus, mitochondria, early and late endosomes) ( Supplementary Fig. S2 ). Furthermore, cell internalization ( Fig. 1g-h ) was not dependent on species (mouse or human, respectively), transformation status (non-malignant or malignant cells), or tumour type (carcinoma (Lewis lung carcinoma), leukaemia (K562), lymphoma (Rauscher murine leukaemia virus antigen), melanoma (B16F10), or sarcoma (KS)). These results show that pen-display mediates the internalization of phage particles into mammalian cells independently of a cell surface receptor, and the internalized particles in the cytosol remain intact, viable and functional within mammalian cells. Therefore, it appeared possible to target a specific organelle, or generate random peptide iPhage libraries to screen for iHoPe in living cells ( Fig. 2a ) with this systematic approach. 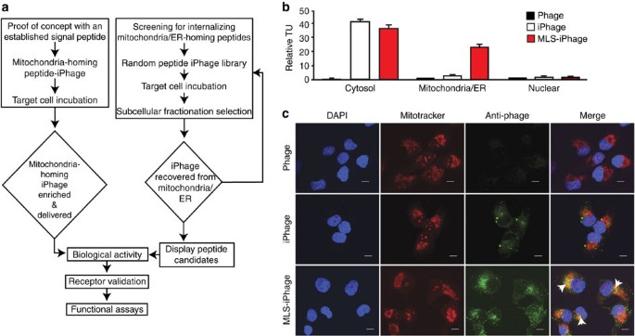Figure 2: Systematic approach for mammalian organelle targeting. (a) Organelle targeting and random peptide iPhage library selection flow diagram. (b) Phage displaying the mitochondrial localization signal of cytochrome c oxidase (MLS-iPhage) in the pIII protein is enriched in the mitochondria/ER fraction. Cytosol and nuclear fractions served as internalizing and negative controls, respectively. Bars represent mean values for TU recovered from the mitochondria/ER fraction±s.e.m., from triplicates. (c) Confocal fluorescence microscopy analysis of KS1767 cells exposed to parental phage, iPhage and MLS-iPhage. Intracellular localization was revealed by anti-rabbit Alexa Fluor 488, orange-Mitotracker, and DAPI counterstaining. Scale Bar, 10 μm. Arrows indicate signal co-localization. Figure 2: Systematic approach for mammalian organelle targeting. ( a ) Organelle targeting and random peptide iPhage library selection flow diagram. ( b ) Phage displaying the mitochondrial localization signal of cytochrome c oxidase (MLS-iPhage) in the pIII protein is enriched in the mitochondria/ER fraction. Cytosol and nuclear fractions served as internalizing and negative controls, respectively. Bars represent mean values for TU recovered from the mitochondria/ER fraction±s.e.m., from triplicates. ( c ) Confocal fluorescence microscopy analysis of KS1767 cells exposed to parental phage, iPhage and MLS-iPhage. Intracellular localization was revealed by anti-rabbit Alexa Fluor 488, orange-Mitotracker, and DAPI counterstaining. Scale Bar, 10 μm. Arrows indicate signal co-localization. Full size image Targeting mitochondria with a localization signal peptide To test whether a defined localization signal peptide displayed by iPhage would target a distinct cellular compartment, we produced an iPhage construct carrying the mitochondria localization signal (MLS), and used this construct to validate the predicted intracellular trafficking of targeted iPhage particles [38] . First, we confirmed that both iPhage and MLS-iPhage were equally efficiently internalized compared with the negative control (parental phage) as observed in the cytosol fraction ( Fig. 2b ). Indeed, MLS-iPhage was detected and enriched by transducing unit (TU) recovery specifically within their corresponding organelle-targeted fraction compared with the nuclear fraction ( Fig. 2b ), and demonstrated by confocal microscopy ( Fig. 2c ). To minimize or eliminate the possibility of an off-target effect, we repeated this proof-of-concept experiment with reduced Mitotracker concentration (fivefold less) and/or shorter incubation time (twofold less); we observed similar target results ( Supplementary Fig. S3 ). Moreover, co-localization index analysis revealed that MLS-iPhage co-localizes to mitochondria tenfold more compared with non-targeted-iPhage particles and 1,000-fold more compared with parental phage ( Supplementary Fig S4 ). Finally, transmission electron microscopy studies revealed that cells treated with MLS-iPhage and the controls (parental and non-targeted-phage) showed MLS-iPhage have clearly entered the target cells, and bound to the mitochondria membrane, but it remains to be determined if they penetrate the organelle under the experimental conditions used; future studies should shed light on whether the sheer size of phage particles or other attributes might preclude or mediate entry into mitochondria. We concluded that iPhage constructs displaying ligand-directed signal peptides penetrated mammalian cells, reached an intracellular equilibrium, and targeted specific compartments within mammalian cells. iPhage library screening yields a new ligand receptor Having demonstrated targeting with a defined intracellular signal peptide, we attempted to identify iHoPe sequences that disrupt cellular viability as a convenient readout for biological activity. Thus, we reasoned that targeting of organelles such as mitochondria and endoplasmic reticulum (ER) would likely be the most suitable way to select and identify candidate pathways involved in cell death [39] . We constructed a random peptide iPhage library [that is, pen displayed on rpVIII and the combinatorial motif arrangement X 4 YX 4 (X, any residue; Y, tyrosine) displayed on pIII] and selected it on live KS1767 cells ( Fig. 3a ). After 24 h, we isolated the mitochondria/ER-enriched fraction and recovered the pool of iPhage through infection of host E. coli . After three rounds of selection, we observed an enrichment of different iPhage clones in the subcellular fraction ( Fig. 3b ). DNA sequencing and bioinformatic analysis revealed a large amount of single peptide iPhage clones in the mitochondria/ER-enriched fraction. Next, we randomly selected ten peptide-iPhage clones and tested their biological activity (disruption of cell viability). The KS1767 cell line was starved overnight and was incubated with each peptide-iPhage clone; as negative control we used insertless parental iPhage in complete MEM media. One should note that the concentration of each peptide-iPhage clone (that is, 10 9 TU per 100 μl) corresponds to only ~60 n M of peptide—an extremely low molar concentration if compared with the amount of synthetic peptide utilized in subsequent cell death experiments (30 μM). After 24 h, we observed morphological alterations and reduced cellular viability only with the YKWYYRGAA-iPhage clone ( Fig. 3c-e ). 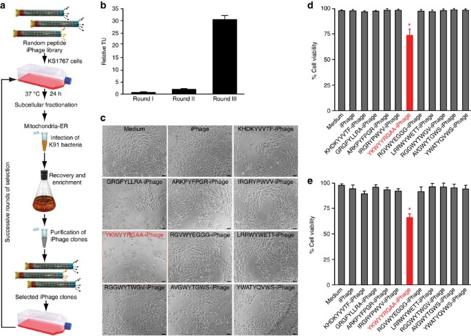Figure 3: Synchronous selection of a random peptide iPhage library is enriched in the mitochondria/ER fraction. (a) Systematic approach of selection in live KS1767 cells. (b) Phage enrichment after three rounds of selection. Bars represent mean values for phage TU recovered from the mitochondria/ER enriched fraction±s.e.m., from triplicates. (c) Bright-field microscopy of KS1767 cells infected with different peptide-iPhage clones selected from the mitochondria/ER fraction. Scale bar, 100 μm. Cell viability was measured using two independent methods (d) WST-1 and (e) MTT assays. Bars represent mean values of cell viability±s.e.m., from triplicates. The symbol * indicates significant reduction of cell viability (P<0.02). Data were statistically analysed by Student'st-test. Figure 3: Synchronous selection of a random peptide iPhage library is enriched in the mitochondria/ER fraction. ( a ) Systematic approach of selection in live KS1767 cells. ( b ) Phage enrichment after three rounds of selection. Bars represent mean values for phage TU recovered from the mitochondria/ER enriched fraction±s.e.m., from triplicates. ( c ) Bright-field microscopy of KS1767 cells infected with different peptide-iPhage clones selected from the mitochondria/ER fraction. Scale bar, 100 μm. Cell viability was measured using two independent methods ( d ) WST-1 and ( e ) MTT assays. Bars represent mean values of cell viability±s.e.m., from triplicates. The symbol * indicates significant reduction of cell viability ( P <0.02). Data were statistically analysed by Student's t -test. Full size image Having shown that MLS-iPhage targets its respective organelle, and the combinatorial selection of YKWYYRGAA-iPhage in mitochondria/ER fraction, we next evaluated the ability of iPhage particles to compete against non-targeted-iPhage particles. First, we show that iPhage particles displaying an organelle-targeting peptide (that is, MLS-iPhage and YKWYYRGAA-iPhage) were selectively enriched in the mitochondria/ER fraction even in the presence of a 10,000-fold molar excess of non-targeted-iPhage particles ( Supplementary Fig. S5 ). Next, to rule out the possibility that particle selection might simply be an artefact (that is, phage binding after the cell fractionation process), we compared an immediate versus a 24-h post-incubation phage-cell fractionation. We observed that iPhage clones (that is, MLS and YKWYYRGAA) were enriched in the respective organelle fraction after overnight post-incubation compared with immediate cell fractionation ( Supplementary Fig. S6 ). Moreover, we detected high amounts of phage in the cytosol when the cell lysate was immediately fractionated compared with fractionation 24 h after incubation ( Supplementary Fig. S6 ), a result indicative of an intracellular steady-state equilibrium. Taken together, these results show that MLS-iPhage and YKWYYRGAA-iPhage particles are retained in the mitochondria/ER fraction irrespective of a competing non-targeted-iPhage, and that they target organelles before cell fractionation. Finally, internalizing versions of the YKWYYRGAA peptide and controls were generated through carboxy-terminal chemical fusions to pen (Merrifield synthesis) and were subsequently evaluated for their intracellular entry and biological activity. RPL29 is a receptor for the internalizing YKWYYRGAA peptide We used affinity chromatography to purify candidate receptors for the YKWYYRGAA peptide and subsequently probed the eluted and immobilized fractions for specific binding of iPhage displaying this ligand peptide ( Fig. 4a ). SDS–PAGE identified a single protein with a relative molecular weight (Mr) of 22,000 Da only in target fraction number 43. Mass spectrometry revealed peptides corresponding unequivocally to the RPL29 ( Fig. 4b ). 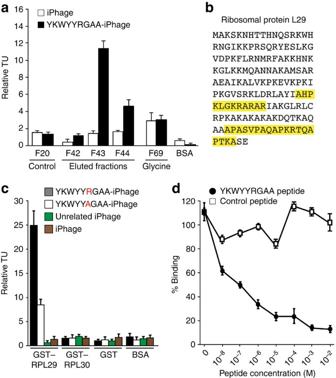Figure 4: RPL29 is the receptor for the internalizing YKWYYRGAA peptide. (a) Phage-binding assay on fractions from YKWYYRGAA affinity chromatography. Fractions were immobilized in a 96-well plate. Insertless iPhage and BSA were used as negative controls. Phage binding assays were run in triplicate; bars represent mean values for phage TU recovered from immobilized proteins±s.e.m., from triplicates. (b) RPL29 was identified by mass spectrometry. Amino acids in yellow represent the peptides detected by mass spectrometry. (c) Phage binding to immobilized GST–RPL29 and GST–RPL30 fusion proteins. BSA or GST alone was used as negative controls. Bars represent mean values for phage TU recovered from immobilized proteins±s.e.m., from triplicates. (d) Binding of the YKWYYRGAA-phage to RPL29 was inhibited with the corresponding synthetic peptide. Bars represent mean±s.e.m., from triplicates. Figure 4: RPL29 is the receptor for the internalizing YKWYYRGAA peptide. ( a ) Phage-binding assay on fractions from YKWYYRGAA affinity chromatography. Fractions were immobilized in a 96-well plate. Insertless iPhage and BSA were used as negative controls. Phage binding assays were run in triplicate; bars represent mean values for phage TU recovered from immobilized proteins±s.e.m., from triplicates. ( b ) RPL29 was identified by mass spectrometry. Amino acids in yellow represent the peptides detected by mass spectrometry. ( c ) Phage binding to immobilized GST–RPL29 and GST–RPL30 fusion proteins. BSA or GST alone was used as negative controls. Bars represent mean values for phage TU recovered from immobilized proteins±s.e.m., from triplicates. ( d ) Binding of the YKWYYRGAA-phage to RPL29 was inhibited with the corresponding synthetic peptide. Bars represent mean±s.e.m., from triplicates. Full size image To confirm the candidate receptor RPL29 as a target for the internalized YKWYYRGAA peptide, we generated a recombinant glutathione S -transferase (GST) fusion with RPL29 and performed binding assays with the YKWYYRGAA-displaying iPhage construct. Consistently, the YKWYYRGAA-displaying iPhage bound to RPL29 but not to control proteins that included a closely related recombinant GST–RPL30 fusion ( Fig. 4c ). Moreover, YKWYYRGAA, but not controls, mediated concentration-dependent inhibition of binding ( Fig. 4d ). Disruption of RPL29 promotes apoptosis induced by a caspase activation pathway in mammalian cells [40] . Therefore, we asked whether the YKWYYRGAA-pen peptide would disrupt RPL29 function and promote cell death. Cell viability assays revealed that YKWYYRGAA-pen, but not control ( Fig. 5a ) or non-conjugated admixtures of pen plus YKWYYRGAA peptides ( Supplementary Fig. S7 ), reduced cell survival; these results were not dependent on transformation status (non-malignant versus malignant cells), species of origin (mouse versus human), or pathological tumour cell type (carcinoma, leukaemia, lymphoma, melanoma, or sarcoma), data suggestive of a general cellular mechanism of cell death ( Supplementary Fig. S8 ). We first analysed the cell surface expression of the established apoptotic marker phosphatidylserine. KS1767 cells were incubated with synthetic YKWYYRGAA-pen, pen alone, or YKWYYRGAA, and were stained with annexin V-fluorescein isothiocyanate (FITC), an early cell death marker. After 6 h, fluorescence-activated cell sorting and fluorescence microscopy revealed that most cells treated with YKWYYRGAA-pen had undergone cell death ( Fig. 5b,c ). To show activation of the intracellular apoptotic pathways, we evaluated the processing of caspase-7 and caspase-9 from inactive zymogen to active protease and observed caspase activation only in the presence of YKWYYRGAA-pen ( Fig. 5d ). Moreover, we detected histone-associated DNA fragments in the cytosol of cells treated only with the YKWYYRGAA-pen peptide; these results suggest that chromatin fragmentation is activated by YKWYYRGAA-pen peptide via RPL29 ( Fig. 5e ). To understand the molecular mechanism(s) of cell death in this new experimental system, we subsequently evaluated biochemical markers related to autophagy and necrosis. In addition to apoptosis, we observed that the marker beclin-1 was upregulated only in cells exposed to YKWYYRGAA-pen peptide, a result suggestive of specific activation of an autophagy-dependent pathway ( Fig. 5f ). Finally, we also investigated cellular necrosis by means of extracellular release of the high mobility group protein B1 (HMGB1). We detected HMGB1 in the supernatant of cells treated only with YKWYYRGAA-pen, a result indicative of necrosis activation pathway ( Fig. 5g ). Taken together, these results show that YKWYYRGAA-pen activates different molecular pathways including apoptosis, autophagy, and necrosis and suggest a complex mammalian cell death mechanism ultimately resulting in morphological alterations consistent with a late stage phenomena illustrated in KS1767 cells by transmission electron microscopy ( Fig. 5h ). After 6 h with the control peptides YKWYYRGAA or pen, the cells remained morphologically normal; in contrast, over 90% of the cells treated with YKWYYRGAA-pen showed the classical morphological signs of cell death (for example, cytoplasmic vacuoles, swollen mitochondria, and chromatin condensation). Notably, during the cell death process, we observed an increasingly translucent cytoplasm, swelling of organelles, and condensation of nuclear chromatin into small, irregular, circumscribed patches through different time points (that is, 0.5, 1 2, and 4 h); these findings were only observed in cells treated with YKWYYRGAA-pen peptide ( Fig. 6a ). We noticed normal and normal-vesicular mitochondria as early as 30 min. However, at 1–2 h, most of the mitochondria showed vesicular-swollen and swollen forms on exposure to the YKWYYRGAA-pen peptide ( Fig. 6b ). These initial functional and morphologic studies indicate that the internalizing RPL29-binding YKWYYRGAA peptide simultaneously activates several mammalian cell death pathways. 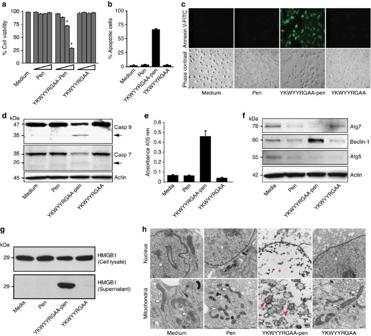Figure 5: The internalizing YKWYYRGAA peptide activates cell death via ribosomal protein L29. (a) Cell viability is reduced on exposure of YKWYYRGAA-pen, relative to complete media, pen, and YKWYYRGAA peptide (1, 3, 10 and 30 μM). The symbol * indicates significant reduction of cell viability (P<0.001; Student'st-test). The MTT assay was performed in triplicate. Bars represent mean±s.e.m. (b) Internalization of YKWYYRGAA peptide induces mammalian cell death. Fluorescence-activated cell sorting of annexin V-FITC-positive cells (apoptotic cells). KS1767 cells were treated with peptides at 30 μM for 6 h at 37 °C. Bars represent mean±s.e.m., from triplicates. (c) Annexin V-FITC binds to translocated phophatidylserine on the plasma membrane of cells treated with YKWYYRGAA-pen. Control, pen, and YKWYYRGAA-treated cells did not translocate the apoptotic marker. Scale bar, 100 μm. (d) The internalizing YKWYYRGAA peptide activates the caspases in the human cell line KS1767. Immunoblotting shows cleavage of caspase-7 (Casp 7) and -9 (Casp 9). Actin served as a loading control. Arrows indicate the caspase fragments. (e) Histone-associated DNA fragments are detected only in cells treated with YKWYYRGAA-pen peptide. DNA fragmentation was detected with the Cell death detection ELISA plus kit (Roche). Bars represent mean±s.e.m., from triplicates. (f) Beclin-1 is upregulated after YKWYYRGAA-pen peptide treatment. Beclin 1, autophagy related protein (atg) 5, and atg-7 expression were detected by western blot. (g) Actin served as a loading control YKWYYRGAA-pen induced the translocation of the high-mobility group protein B1 (HMGB1) into the extracellular environment. KS1767 cells were treated with different peptides at 30 μM or with media as indicated. (h) Normal mitochondria change to vesicular form, and the matrix swells (red arrows). Chromatin condensation and fragmentation (red asterisk) are observed only in KS1767 cells exposed to YKWYYRGAA-pen. Normal mitochondria (white arrows) and nuclei (white asterisks) are observed in control-untreated, pen-treated, and YKWYYRGAA-treated cells. Scale bar, 500 nm. Figure 5: The internalizing YKWYYRGAA peptide activates cell death via ribosomal protein L29. ( a ) Cell viability is reduced on exposure of YKWYYRGAA-pen, relative to complete media, pen, and YKWYYRGAA peptide (1, 3, 10 and 30 μM). The symbol * indicates significant reduction of cell viability ( P <0.001; Student's t -test). The MTT assay was performed in triplicate. Bars represent mean±s.e.m. ( b ) Internalization of YKWYYRGAA peptide induces mammalian cell death. Fluorescence-activated cell sorting of annexin V-FITC-positive cells (apoptotic cells). KS1767 cells were treated with peptides at 30 μM for 6 h at 37 °C. Bars represent mean±s.e.m., from triplicates. ( c ) Annexin V-FITC binds to translocated phophatidylserine on the plasma membrane of cells treated with YKWYYRGAA-pen. Control, pen, and YKWYYRGAA-treated cells did not translocate the apoptotic marker. Scale bar, 100 μm. ( d ) The internalizing YKWYYRGAA peptide activates the caspases in the human cell line KS1767. Immunoblotting shows cleavage of caspase-7 (Casp 7) and -9 (Casp 9). Actin served as a loading control. Arrows indicate the caspase fragments. ( e ) Histone-associated DNA fragments are detected only in cells treated with YKWYYRGAA-pen peptide. DNA fragmentation was detected with the Cell death detection ELISA plus kit (Roche). Bars represent mean±s.e.m., from triplicates. ( f ) Beclin-1 is upregulated after YKWYYRGAA-pen peptide treatment. Beclin 1, autophagy related protein (atg) 5, and atg-7 expression were detected by western blot. ( g ) Actin served as a loading control YKWYYRGAA-pen induced the translocation of the high-mobility group protein B1 (HMGB1) into the extracellular environment. KS1767 cells were treated with different peptides at 30 μM or with media as indicated. ( h ) Normal mitochondria change to vesicular form, and the matrix swells (red arrows). Chromatin condensation and fragmentation (red asterisk) are observed only in KS1767 cells exposed to YKWYYRGAA-pen. Normal mitochondria (white arrows) and nuclei (white asterisks) are observed in control-untreated, pen-treated, and YKWYYRGAA-treated cells. Scale bar, 500 nm. 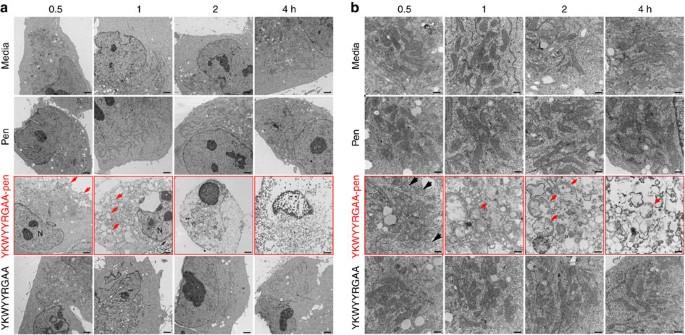Figure 6: The YKWYYRGAA-pen peptide induces ultrastructural alterations leading to cell death. (a) Electron microscopy analysis of KS1767 cells untreated (media) and treated with peptides (30 μM) at different time points (0.5, 1, 2, and 4 h). The cells treated only with the YKWYYRGAA-pen peptide suffered ultrastructural alterations as early as 30 min; the plasma membrane and the cytoplasm were extensively dismantled (red arrows) compared with cells treated with peptide controls or media. Scale bar, 2 μm. (b) Intracellular compartments analysis by transmission electron microscopy shows normal-vesicular (black arrow) to swollen mitochondria (red arrow), such structural alterations were only observed in KS1767 cells treated with YKWYYRGAA-pen peptide (30 μM). Normal mitochondria were observed in KS1767 cells treated with control peptides (30 μM) and media. Scale bar, 500 nm. Full size image Figure 6: The YKWYYRGAA-pen peptide induces ultrastructural alterations leading to cell death. ( a ) Electron microscopy analysis of KS1767 cells untreated (media) and treated with peptides (30 μM) at different time points (0.5, 1, 2, and 4 h). The cells treated only with the YKWYYRGAA-pen peptide suffered ultrastructural alterations as early as 30 min; the plasma membrane and the cytoplasm were extensively dismantled (red arrows) compared with cells treated with peptide controls or media. Scale bar, 2 μm. ( b ) Intracellular compartments analysis by transmission electron microscopy shows normal-vesicular (black arrow) to swollen mitochondria (red arrow), such structural alterations were only observed in KS1767 cells treated with YKWYYRGAA-pen peptide (30 μM). Normal mitochondria were observed in KS1767 cells treated with control peptides (30 μM) and media. Scale bar, 500 nm. Full size image The signal hypothesis and the existence of intracellular ZIP codes are both well-recognized fundamental concepts in cell biology [41] , [42] , [43] . However, in contrast to ligand-directed targeting of cell membranes in vitro [6] , [26] or in vivo [1] , [2] , [3] , [44] , [45] , combinatorial phage display-based technology has not yet been extended to the analysis of intracellular organelles and signalling or metabolic pathway targets in live cells. We have approached this methodological gap through the display of established internalizing peptides [46] , [47] . We chose pen, an internalizing peptide, which is derived from the homeodomain of the Drosophila melanogaster antennapedia protein [21] , [36] . We have shown that expression of pen as a fusion recombinant protein on the major capsid rpVIII allows passage into cultured mammalian cells of viable, functional internalizing phage (named iPhage), without the participation of cell surface receptors. Fusing a known signal peptide [38] to the phage pIII protein directs intact iPhage particles to the predicted intracellular location; the simultaneous display of a random peptide on iPhage results in the selection and differential distribution of iPhage among the subcellular compartments, and peptides displayed in the iPhage particles can mimic their function with synthetic peptide counterparts. We further demonstrate the power of this methodology by identifying an iHoPe and its corresponding receptor mediating mammalian cell death. RPL29 is a conserved protein involved in the assembly of the 60S ribosomal subunit, and studies in yeast have demonstrated that inactivation or mutation of the RPL29 gene retards protein synthesis [48] . RPL29 gene inactivation in mice showed an alteration in the cell cycle, and as a result, RPL29-null newborn pups were reduced to half in size [49] . One may speculate that YKWYYRGAA-pen disrupts RPL29 function in ribosome assembly and protein synthesis, and thereby promotes cell death. Notably, the productive assembly of YKWYYRGAA-displaying iPhage particles indicates that this peptide is non-toxic to host bacteria and therefore does not appear to affect bacterial ribosomes, but rather targets eukaryotic ribosomes selectively. The YKWYYRGAA-pen peptide shows a remarkable activation of multiple mammalian cell death pathways at the biochemical level including apoptosis, autophagy and necrosis [50] , [51] , [52] , [53] . However, future studies will be required to dissect the inherent, biologically complex death mechanism of the YKWYYRGAA-pen peptide via RPL29 in mammalian cells beyond the scope of this initial communication. The relevance of subcellular targeting for drug delivery to improve drug efficiency, via the release of compounds within organelles, has recently been recognized [54] . The iPhage technology originally reported here has not only the potential for subcellular delivery, but might also unveil iHoPe sequences relevant to intracellular trafficking in live cells. Finally, this internalizing strategy could also be combined with adeno-associated virus phage--based vectors for improved mammalian cell expression [55] . In summary, this new combinatorial approach employing internalizing peptides enables ligand-directed discovery of signal peptides and targeting of organelles or molecular pathways within live cells, with potential applications ranging from cell biology to drug development. Reagents The following antibodies were obtained from commercial sources: anti-bacteriophage antibody (1:1000, Sigma), anti-caspase-7, anti-caspase-9, anti-atg-5, anti-atg-7, anti-beclin-1 (1:2000, Cell Signaling Technology), anti-HMG-B1 (1:2000, Millipore), anti-actin antibody (1:5000, Novus Biologicals), anti-rabbit Cy3, anti-mouse FITC, anti-goat FITC (1:300, Zymed), anti-mouse HRP (1:5000, Bio-Rad), Alexa Fluor 488 goat anti-rabbit (1:500, Invitrogen), goat and mouse pre-immune sera (1:300, Jackson Immunoresearch). The following fluorescence probes were used: 4,6-diamidino-2-phenylindole (DAPI) (Vector Laboratories), ProLong Gold antifade reagent, Orange MitoTracker (Invitrogen), and annexin V-FITC (BD Biosciences). Molecular biology reagents included restriction enzymes (New England Biolabs and Roche), T4 DNA ligase (Invitrogen), Taq DNA polymerase (Promega, Stratagene and Invitrogen); gel extraction, PCR purification, and plasmid isolation kits (Qiagen), isopropyl b- D -1-thiogalactopyranoside (IPTG; Fisher Scientific). We used commercial recombinant ribosomal protein L30 (RPL30; Novus). All the synthetic peptides were produced to our specifications (PolyPeptide Laboratories). Cell culture Human Kaposi sarcoma (KS1767) cells were maintained in MEM containing 10% FBS, MEM-vitamins, non-essential amino acids, penicillin G (100 units), streptomycin SO 4 (100 mg ml −1 ), and 2.7 mM. L -glutamine (Invitrogen) at 37 °C in a 5% CO 2 -humidified incubator. Phage internalization assay For mammalian cell internalization, KS1767 cells were grown in 8-well tissue-chamber slides and incubated with 10 9 TU of iPhage, mutant iPhage, or parental insertless phage in MEM containing 1% bovine serum albumin (BSA) at 37 °C. After 24 h of incubation, cell membrane-bound phage was removed by acidic washing (20 mM glycine, pH 2.3). Cells were washed with PBS and fixed with 4% paraformaldehyde in PBS at room temperature for 15 min. After washes with PBS, fixed cells were rendered permeable with PBS containing 0.1% Triton X-100 (Sigma), blocked with PBS containing 1% BSA, and incubated with anti-bacteriophage (1:200 dilution) in PBS containing 1% BSA for 2 h at room temperature. Next, Cy3-conjugated anti-rabbit (1:200 dilution) was added, and incubated at room temperature for 1 h. Finally, cells were washed with PBS, fixed with PBS containing 4% paraformaldehyde, mounted in the presence of DAPI (Invitrogen), and visualized under a fluorescence or confocal microscope. Generation of the iPhage peptide display library To generate iPhage constructs, we transformed the M13-derived vector f88-4 (AF218363) into MC1061 E. coli . Single colonies were selected on Luria-Bertani (LB) agar plates with tetracycline (40 mg ml −1 ) and streptomycin (50 mg ml −1 ) and cultured overnight. Each plasmid DNA was first isolated by standard plasmid purification kit (Siegen) and was subsequently re-purified through a CsCl gradient. Next, annealed oligonucleotides encoding the penetratin peptide, sense 5′-cacaagctttgccaacgtccctc gacagataaagatttggttccaaaacggcgcatgaagtggaagaagcctgcagcaca-3′; antisense 5′-tgtgc tgcaggcttcttc cacttcatgcgccggttttggaaccaaatctttatctgtcgagggacgttggcaaagcttgtg-3′), and f88-4 plasmid were digested with Hind III and Pst I restriction endonucleases. DNA fragments were gel-purified (Qiagen) and ligated at various vector: insert molar ratios. Restriction enzyme-digested and sequence-verified individual clones were electroporated into MC1061 E. coli ; iPhage particles were cultured in LB media containing 1 mM IPTG, tetracycline (40 mg ml −1 ), and streptomycin (50 mg ml −1 ), and were purified by the polyethylene glycol-NaCl method [56] . To produce an iPhage library displaying the peptide insert in the minor pIII coat protein (general arrangement X 4 YX 4 ), we fused the iPhage construct (described above) and fUSE5 genomes to create a chimeric vector. Both plasmids were digested with BamH I and Xba I restriction enzymes, and the products were resolved on a 0.8% agarose gel. A DNA fragment of 3,925 bp from fUSE5 (containing the rpIII) and another 5,402 bp fragment of iPhage (containing the rpVIII) were gel-purified and ligated overnight at 16 °C. Ligated products were precipitated in ethanol and electroporated into MC1061 E. coli ; these bacteria were plated on LB-agar and selected with tetracycline and streptomycin. Next, we performed a CsCl plasmid purification of the iPhage/fUSE5 chimeric vector, which was digested with Sfi I restriction endonuclease. In parallel, we performed a PCR amplification of the degenerate oligonucleotide (5′-cactcggccgacggggctnnknnknnknnktatnnk nnknnknnkggggccgctggggccgaa-3′) insert sequence with Bgl I restriction sites at both DNA ends [57] . The PCR products were purified on Qiagen columns, digested with Bgl I, and gel-purified. Sfi I-linearized iPhage/fUSE5 and double-stranded oligonucleotide inserts were prepared for large-scale ligations. After overnight incubation, ligated products were precipitated in ethanol and reconstituted in sterile water. We performed over 250 electroporations in MC1061 E. coli and transferred them into super optimal broth with catabolite repression medium at 37 °C for 1 h. Finally, the bacterial culture was amplified in LB medium (4 l) containing 1 m M IPTG, tetracycline (40 mg ml −1 ), and streptomycin (50 mg ml −1 ); phage particles were recovered to yield an X 4 YX 4 -iPhage display library. iPhage library intracellular selection KS1767 cells were incubated with 5×10 11 TU of the X 4 YX 4 iPhage library overnight at 37 °C. The next day, cells were washed extensively with pre-warmed PBS and were subsequently detached with trypsin. Cells were washed with ice-cold PBS, incubated with hypotonic buffer (10 mM NaCl, 1.5 mM MgCl 2 , 10 mM Tris–HCl (pH 7.5)) for 15 min, and placed in a standard Dounce homogenizer to disrupt cell membranes. Next, we added stabilization buffer (525 mM mannitol, 175 nM sucrose, 2.5 mM EDTA (pH 7.5), and 12.5 mM Tris–HCl (pH 7.5)). The organelle suspension obtained was centrifuged at 1,300 g for 5 min at 4 °C; the supernate was transferred to a new tube, and centrifuged at 17,000 g for 15 min; this pellet contained the mitochondria-/ER-enriched fraction. The subcellular fraction-bound phage population was recovered through infection of log-phase k91kan E. coli for 1 h at room temperature. Serial dilutions of the infected bacteria were plated on LB plates containing tetracycline (40 mg ml −1 ) and kanamycin (100 mg ml −1 ) to determine the recovery phage titre. In addition, infected bacteria were grown overnight in LB containing tetracycline and kanamycin, and phage was recovered by polyethylene glycol/NaCl precipitation [56] , [57] . After 3 rounds of selection, 96 bacterial colonies from each round were randomly selected for DNA sequencing. Confocal imaging The cells were imaged with an inverted Olympus FV1000 (Olympus, Center Valley, Pennsylvania, USA) laser scanning confocal microscope using a ×60 O3 PLAPO oil objective. The imaging and 3D reconstruction was performed by taking a series of horizontal scans through the cells, arranged as a vertical stack/z-stack by means of image analysis software ( FV1000 version 1.6, Olympus Inc). Optical sections were acquired at 0.44 μm intervals, with an imaging stack consisting of 22 optical sections. The image size was an 800×800 pixel matrix per image (132×132 μm) with a colour depth of 12 bits per pixel. In this study, we used the UV LD405 nm laser (Olympus America, Center Valley, Pennsylvania, USA) as well as the Argon ion 488 nm and green HeNe 543 nm lasers (Melles Griot, Albuquerque, New Mexico,USA) and suitable filter sets. Binding assay and ligand receptor purification By coupling the selected synthetic peptide to a Sepharose column (Carboxy-link kit, Pierce) and exposing the columns to KS1767 cell-derived lysates, we purified a candidate receptor. After extensive washing, the receptor was eluted with the corresponding competitive peptide at a concentration of 5 mM. Eluted fractions were analysed by absorbance (optical density at 280 nm), dialysed, and concentrated at 4 °C. Equal amounts of protein (5 μg per well in 50 μl PBS) were immobilized on a 96-well plate overnight at 4 °C. Wells were washed twice with PBS, blocked with PBS containing 2% BSA for 2 h at room temperature, and incubated with targeted iPhage or parental insertless iPhage (10 9 TU each) in 50 μl PBS containing 0.1% BSA. After 2 h at room temperature, wells were washed ten times with PBS, and each phage population was recovered by host bacterial infection. Cell death assays KS1767 cells grown in 48-well plates were maintained for 24 h in non-supplemented MEM. The medium was subsequently supplemented with 10% FBS plus each respective test peptide. Cellular viability was assessed by measurement of cellular metabolism by the MTT (Roche), and WST-1 (Roche) assays at 37 °C, according to standard protocols. Staining for annexin V (Clontech) was performed to monitor early stages of apoptosis. KS1767 cells grown in 8-well slide chambers were incubated with the peptides for 6 h. Next, cells were incubated with annexin V-FITC, washed, and analysed under a fluorescence microscope. For flow cytometry analysis, cells were detached and washed twice with cold PBS and then resuspended in binding buffer (Clontech) at a concentration of 10 6 cells ml −1 . We transfer 100 μl of the solution to a 5-ml culture tube and added annexin-V-FITC and incubated for 15 min room temperature. The cells were washed twice with binding buffer and analysed by flow cytometry. Statistical analysis Student's t -tests were used for statistical analysis as indicated. How to cite this article: Rangel, R. et al . Combinatorial targeting and discovery of ligand-receptors in organelles of mammalian cells. Nat. Commun. 3:788 doi: 10.1038/ncomms1773 (2012).